Genome-wide search for exonic variants affecting translational efficiency The search for expression quantitative trait loci has traditionally centred entirely on the process of transcription, whereas variants with effects on messenger RNA translation have not been systematically studied. Here we present a high-throughput approach for measuring translational cis- regulation in the human genome. Using ribosomal association as proxy for translational efficiency of polymorphic messenger RNAs, we test the ratio of polysomal/non-polysomal messenger RNA level as a quantitative trait for association with single nucleotide polymorphisms on the same messenger RNA transcript. We identify one important ribosomal distribution effect, from rs1131017 in the 5′-untranslated region of RPS26 , that is in high linkage disequilibrium with the 12q13 locus for susceptibility to type 1 diabetes. The effect on translation is confirmed at the protein level by quantitative western blots, both ex vivo and after in vitro translation. Our results are a proof-of-principle that allelic effects on translation can be detected at a transcriptome-wide scale. Genetic effects on gene expression or expression quantitative trait loci (eQTLs), are common in the human genome [1] , [2] , [3] , [4] , [5] , [6] , [7] and their elucidation is critical for understanding human genetic diseases [8] , [9] , [10] , especially those with complex-trait inheritance. Previous genome-wide eQTL searches have focused exclusively on the levels of steady-state messenger RNA, for the discovery of variants modulating transcription or RNA stability. However, as the biological effect of altering expression levels of most genes depends on allelic protein levels, the potential effect of polymorphic RNA on translation may be equally important and is required to complete the picture [11] , [12] . DNA sequence variants can affect translational efficiency through different mechanisms [12] : (1) at the 5′-untranslated region (UTR), a variant can abolish or create a upstream translation-initiation codon or open reading frame [13] , [14] , [15] , or change an internal ribosome entry site by loss-of-function [16] or gain-of-function [17] ; (2) at the translation start site, a mutation can change the highly conserved Kozak sequence gccRCCAUGG [18] , [19] ; (3) at a splice-site of the exon–intron junction, a mutation can cause the production of an mRNA isoform with missing 5’-UTR functional elements [20] ; (4) at the 3'-UTR, a mutation changing the upstream core polyadenylation signal sequence consensus sequence, the hexamer AAUAAA, may lead to alternative mRNA isoforms with different 3′-UTR structure and poly(A) tail, and therefore differential translational properties [21] , [22] , [23] . Most of these examples have been demonstrated with mutations causing rare monogenic diseases. For common DNA variations, much fewer examples exist. Perhaps the best-known example is the case of a haplotype of synonymous single nucleotide polymorphisms (sSNPs) at the COMT gene encoding the enzyme catechol-o-methyltransferase, which alter the secondary structure of mRNA and the efficiency of protein expression, a probable explanation for their effect on pain sensitivity [24] . In addition, a sSNP may change the translational efficiency on the basis of differential transfer RNA abundance for different codons that shape codon usage [25] , [26] . Evidence of selective pressure [27] indeed suggests a functional role for some sSNPs. To date, the role of common DNA variation on mRNA translation has received little attention, probably because of the obvious methodological limitations of high-throughput quantitative proteomics as compared with oligonucleotide expression microarrays or RNAseq. As a potential remedy for this gap, we undertook this study to examine the feasibility of systematically screening human genetic variants that affect the ribosomal distribution of mRNA, taken as a proxy for translational efficiency. This is based on the principle that efficiently translated mRNAs associate with multiple ribosomes, whereas less active ones associate with fewer or none. We leverage the extensively validated ultracentrifugal method for estimating translational activity based on the sedimentation velocity of mRNA–ribosomal complexes [28] , [29] , [30] , using immortalized lymphoblastoid cell lines (LCLs), a cell type extensively used in functional genomics studies [31] . Genome-wide screening for SNPs with translational effect We studied human immortalized LCLs of 38 parents of the HapMap European families of Utah residents with Northern and Western European ancestry (CEPH Europeans from Utah (CEU)) from the Centre de l’Étude du Polymorphisme Humain (CEPH). A total of 52,737 exonic SNPs in 15,265 autosomal genes with minor allele count ≥5 (that is, MAF≥6.6%) were evaluated (60,425 exonic SNP–gene pairs, Supplementary Data 1 ), setting a Bonferroni threshold of 8.3 × 10 −7 . Because of the common existence of overlapping genes, one SNP may map to two genes at the same time. Among these SNPs, 35,620 (67.5%) were genotyped in HapMap and 17,117 (32.5%) SNPs were detected by the 1000 Genomes Project in 29 of the 38 subjects. The distribution of imputation quality scores of SNPs in the nine samples without the 1,000 genomes genotyping is shown in Supplementary Fig. S1 . Eleven SNPs in six genes met the Bonferroni threshold, whereas 74 SNPs in 29 genes met the false discovery rate (FDR) Q -value<0.1 ( Supplementary Table S1 ). 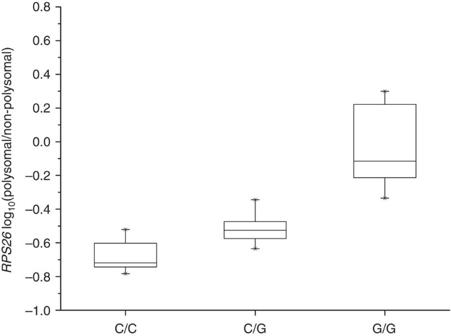Figure 1:RPS26mRNA polysomal/non-polysomal ratio and rs1131017 genotypes. The log-transformed mRNA ratio of normalized signals of polysomal/non-polysomal is associated with the rs1131017 genotypes with high statistical significance (n=38, Spearman rank correlationP=3.79 × 10−13). Error bars represent 25 and 75% percentiles. The G allele of rs1131017 is correlated with higher polysomal/non-polysomal ratio. Among SNPs with Q <0.1, 5′-UTR SNPs were significantly enriched (20.3% versus 9.9%, P =2.78 × 10 −3 ) ( Table 1 ). 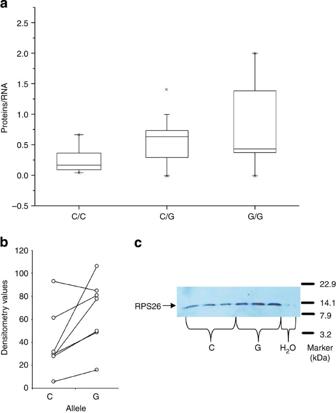Figure 2: Confirmation of translational effects inRPS26at the protein level. (a) RPS26 protein levels byex vivotranslation quantification. The mRNA-normalized protein levels ofRPS26between the three genotypes showed statistically significant correlation (n=36, Student'st-testP=0.005), and the G allele of rs1131017 is correlated with higher protein levels. Error bars represent 25 and 75% percentiles. (b) RPS26 protein levels byin vitrotranslation and immunoblot quantification. Comparison ofRPS26constructs with rs1131017 C/G alleles. Each western blot contained at least three replicates for each allele (C or G). Statistical significance favouring the construct with the G allele was found (pairedt-testP=0.0204). (c) TheRPS26constructs containing different alleles of rs1131017 produced different levels ofRPS26protein. The G allele of rs1131017 produced higher level ofRPS26protein. A representative of seven translation runs is shown. Among the 74 SNPs with FDR<0.1, 4 SNPs are in linkage disequilibrium (LD, r 2 >0.5) with SNPs identified as those associated with disease susceptibility ( Table 2 ). Table 1 SNP functional classifications. Full size table Table 2 SNPs with possible translational cis- regulatory effects and disease association. Full size table To look for alternative splicing as the mechanism of such effects, we intersected the set of our SNPs with a list of 187 splicing quantitative trait loci, discovered by Pickrell et al. [32] using RNA sequencing. We found two overlaps, interestingly, both in highly polymorphic genes of the major histocompatibility complex on 6p21. The first is SNP rs241451, associated with the splicing of the last exon of TAP2 . As our group has previously shown [33] , it creates two transcripts (GenBank Nucleotide Accession codes NM_000544 and NM_018833 ) with completely distinct carboxy terminals and 3′-UTRs, which explains the translational effect. The second one is at HLA-C , where rs7767581 is associated with the splicing of an exon encoding the highly conserved functional α3 domain [34] . Such an overlap is not surprising. If both isoforms encode the same protein, splicing is just one of the mechanisms of polymorphic translational control. Even if the proteins are different, the effect on translation should be factored into the mechanisms by which the locus exerts phenotypic effects. We also found that two of our hits overlapped with eQTLs for steady-state mRNA in LCLs [6] ( http://www.sph.umich.edu/csg/liang/asthma/ ). They involve TAP2 (as shown in our previous report [33] ) and ZNF584 . In both cases, the haplotype associated with higher translational efficiency also has higher mRNA level, which may be related to the ribosome protection of mRNA from endonucleolytic attacks for the actively translated allele [35] . Translational effects in RPS26 at the protein level One of the most significant effects on ribosomal distribution was found in the RPS26 gene ( Fig. 1 ), by a 5′-UTR SNP that is in tight LD with the most significant SNP at the type 1 diabetes risk locus on 12q13 (refs 36 , 37 ). It was chosen for validation at the protein level. Figure 1: RPS26 mRNA polysomal/non-polysomal ratio and rs1131017 genotypes. The log-transformed mRNA ratio of normalized signals of polysomal/non-polysomal is associated with the rs1131017 genotypes with high statistical significance ( n =38, Spearman rank correlation P =3.79 × 10 −13 ). Error bars represent 25 and 75% percentiles. The G allele of rs1131017 is correlated with higher polysomal/non-polysomal ratio. Full size image To confirm that ribosomal distribution does reflect a translational effect at the protein level, we tested the assumption that the mRNA allele found at a higher proportion in the polyribosomal fraction than in the soluble RNA will produce more protein product under the same translational environment. We tested this expectation in the case of allelic effects of rs1131017 on RPS26 protein translation by two independent approaches, that is, protein quantification ex vivo and following in vitro translation of allelic constructs. In ex vivo translation quantification, the RPS26 RNA and the RPS26 protein from 36 LCL samples were quantified and compared based on their genotypes. We compared the mRNA-normalized protein levels of RPS26 between the three genotypes. Statistically significant correlation (Student's t -test P =0.005) was found with the rs1131017genotype ( Fig. 2a ). The ex vivo results show that the mRNA with the G allele of rs1131017 produces significantly more protein, which is concordant with the microarray result. Protein also correlates with the ribosomal distribution ratio, independent of genotype: r = 0.449, correlated samples t -test P =0.028). In the in vitro translation quantification, paired t -test was applied to compare the constructs containing each allele of rs1131017 in seven distinct in vitro translation experiments with each western blot membrane containing at least three replicates of each genotype. We found again that the G allele of rs1131017 showed higher translational efficiency by producing more protein (paired t -test P =0.020) ( Fig. 2b,c ). This observation confirms the ex vivo results, both results showing that the G allele of rs1131017 that was found to be most strongly associated with polysomal distribution is also producing more protein. Figure 2: Confirmation of translational effects in RPS26 at the protein level. ( a ) RPS26 protein levels by ex vivo translation quantification. The mRNA-normalized protein levels of RPS26 between the three genotypes showed statistically significant correlation ( n =36, Student's t -test P =0.005), and the G allele of rs1131017 is correlated with higher protein levels. Error bars represent 25 and 75% percentiles. ( b ) RPS26 protein levels by in vitro translation and immunoblot quantification. Comparison of RPS26 constructs with rs1131017 C/G alleles. Each western blot contained at least three replicates for each allele (C or G). Statistical significance favouring the construct with the G allele was found (paired t -test P =0.0204). ( c ) The RPS26 constructs containing different alleles of rs1131017 produced different levels of RPS26 protein. The G allele of rs1131017 produced higher level of RPS26 protein. A representative of seven translation runs is shown. Full size image RPS26 and type 1 diabetes susceptibility RPS26 maps to a region of Chr12q13.2, which is known to confer type 1 diabetes susceptibility as determined in the genome-wide association studies (GWASs) conducted by the Wellcome Trust Case-Control Consortium, our group, and the Type 1 Diabetes Genetics Consortium (T1DGC) [36] , [37] , [38] , [39] , [40] , [41] , as well as in studies on other autoimmune diseases [42] , [43] . The SNP identified to have a cis -translational effect is in high LD with SNPs tagging T1D genetic susceptibility, that is, rs1701704 (ref. 37 ), rs11171739 (ref. 39 ) and rs2292239 (refs 36 , 40 , 41 ) ( Supplementary Fig. S2 ). The allele with lower translational activity is in LD with the T1D predisposing effect. The G allele interrupts an oligopyrimidine tract, which has a role in translational repression [44] . Because of the availability of microarray technologies for high-throughput transcriptome profiling, numerous eQTL studies on gene transcription have successfully acquired knowledge of the genetic regulation of gene transcription in human diseases. However, no such high-throughput method exists to study genetic regulation of translation genome wide. Despite the rapid progress in proteomics technologies, quantitative assays of proteomics are much more complicated and expensive, and also lack the precision and dynamic range of transcriptome assays. In this study, we created a novel high-throughput approach to discover the genetic effect on mRNA translation using ribosomal association as proxy, to drastically narrow down the range of targets for proteomic validation. Because ribosomal fractionation is costly and labour intensive, we felt that a small pilot study was justified before investing in more powerful sample sizes. Despite the very small sample size and consequent reduced statistical power, we were able to detect 29 genes subject to genetic modulation in cis at the translational level. Nevertheless, 29 represents a much smaller number of translational eQTLs than those found at the transcriptional level. We propose that this is only a matter of statistical power and that these 29 genes represent the ‘tip of the iceberg’, as indicated by the Quantile–Quantile plot ( Supplementary Fig. S3 ). The same approach, applied to hundreds of samples will probably reveal a much larger number of loci, conceivably comparable with that of genetic effects on transcription. Regardless of their actual numbers, the utility of discovering genetic loci affecting translation is enhanced by the ability to easily identify the causal variant as it is constrained to map on the mRNA, whereas transcriptional variants must be sought over genomic regions that are orders of magnitude wider. Aligning our results with GWAS findings, we found 3 of the 29 loci mapping to loci of susceptibility to human diseases. The most interesting example is the ribosomal protein S26 gene ( RPS26 ) at a risk locus for type 1 diabetes and other autoimmune diseases [36] , [37] , [38] , [39] , [40] , [41] , [43] , [45] . The RPS26 SNP rs1131017 identified to have cis -translational effect is in high LD with the genetic markers of T1D and Vitiligo susceptibility. The SNP rs1131017 maps to a 5′ terminal oligopyrimidine tract identified in the mRNAs encoding the ribosomal proteins in mammalia, which has the role of translational repression [44] . Interruption of the terminal oligopyrimidine tract by rs1131017 may thus alleviate the translational repression. The same SNP has been reported to also have a transcriptional effect on the gene, which, however, goes in the opposite direction [6] , [46] . The two opposing effects probably cancel each other, at least partially, which may be consistent with the statistical analysis indicating that the transcriptional effect is probably not causal in this association [47] . However, many transcriptional effects (and, in all likelihood, translational ones) are tissue-specific. It is quite possible that, in some T1D-relevant tissues only one of the two effects modulates expression, in which case this conclusion will need to be re-evaluated. Translational eQTL studies with larger sample sizes will be needed to address this question. In conclusion, the approach developed in this study covers an aspect of functional genomics that has not received much attention so far, and adds an important tool to the evaluation of genetic loci associated with complex disorders. This study screened the human genome systematically for cis -regulation effect on gene translation in LCLs. It is readily expandable to study cell- or tissue-specific genetic effect of gene translation by investigating different cell lines or tissues. Larger sample sizes are likely to reveal a number of effects that rival that of transcriptional effects. Ideally, such questions can be answered by direct quantification of proteins. However, hypothesis-free methodologies for proteome-wide quantification have significant drawbacks [48] , whereas targeted proteomics with selected reaction monitoring now allows sensitive quantification with no need for affinity reagents [49] . Our methodology will be most useful in identifying candidates for confirmation by selected reaction monitoring. The latter can also be used to detect post-translational modifications [50] thus covering all processes by which genetic variation affects gene expression. Cell lines The LCLs were acquired from the Coriell Institute for Medical Research ( http://ccr.coriell.org/Sections/Collections/NHGRI/hapmap.aspx?PgId=266&coll=HG , New Jersey, USA). These LCLs have been genotyped for ~9 million SNPs on autosomes by the HapMap project ( http://www.hapmap.org/ ) and the 1000 Genomes Project (the March 2010 release, http://www.1000genomes.org ). The cells were cultured using RPMI-1640 containing 15% fetal bovine serum (FBS), 1% L-glutamine, 1% penicillin and 1% streptomycin, in a 37 °C 5%CO 2 incubator. The Research Ethics Board of the Montreal Children’s Hospital approved the study. Polyribosome fractionation RNA molecules were fractionated on the basis of the number of ribosomes they were associated with, by ultracentrifugal sedimentation velocity in viscous media (sucrose gradients). The larger aggregates of the more actively translated RNA sediment faster than the smaller aggregates, whereas the RNA that is not associated with ribosomes remains at the top layer [28] , [51] . From each LCL, 1 × 10 8 cells were incubated with 100 μg μl −1 cycloheximide for 5 min at 37 °C to freeze translational activity and then washed with PBS containing 100 μg ml −1 cycloheximide. Cell pellets, collected by centrifugation at 1,000 r.p.m. for 10 min at 4 °C, were lysed with hypotonic polysome lysis buffer (5 mmol l −1 Tris-HCl (pH 7.5), 2.5 mmol l −1 MgCl 2 , 1.5 mmol l −1 KCl, 100 μg ml −1 cycloheximide, 2 mmol l −1 dithiothreitol (DTT), 10% Triton X-100, and 10% sodium deoxycholate). After 2 min of incubation on ice in a prechilled Eppendorf tube, with occasional vortexing, the extracts were centrifuged for 2 mins at 13,000 r.p.m. at 4 °C to remove cellular debris. The supernatant was directly loaded on a 10–50% linear sucrose gradient (20 mmol l −1 HEPES-KOH (pH 7.6), 100 mmol l −1 KCl, 5 mmol l −1 MgCl 2 ) and then centrifuged in a Beckman SW41 rotor for 120 min at 35,000 r.p.m. at 4 °C. As stated earlier, mRNA directing enhanced protein synthesis at many ribosomes simultaneously is expected to be more abundant in the heavier polysome fractions, whereas mRNA subjected to repressed translation should be more abundant in fractions spanning low-number polysomes, monosomes and free ribosomal subunits. Polyribosomal fractions were collected using the Brandel fraction collector (Gaithersburg, Maryland, USA) with real-time monitoring of ultraviolet optical density at 254 nm using an ISCO type 11 optical unit connected with a recorder. There were 24 fractions per cell line. Sample preparation and microarray analysis After the fractions were collected, RNA from each fraction was extracted using TRIzol (Invitrogen, California, USA) followed by the phenol–chloroform purification. The mRNA concentration of each fraction was quantified by slot-blot hybridization using digoxigenin-labelled oligo-dT to quantify poly-A RNA ( Supplementary Figs S4,S5 ). Equal amounts of poly-A RNA (5 ng μl −1 ) from unfractionated RNA, non-polysomal RNA (four fractions before the 80S polysome peak) and polysomal RNA (four fractions after the polysomal fraction peak) of every individual were evaluated for genome-wide expression profiling on the Illumina HumanRef-8 v3.0 Expression BeadChip (Illumina, San Diego, California). The selection of polysome fractions of each individual was based on the real-time optical density detection in the fractionation process. The selection of non-polysomal fraction and the polysomal fraction is illustrated in Figure3 . If the profile of a cell line did not fit the exact pattern, the extraction was repeated. All decisions to repeat were made before the availability of any microarray results. Our quality control process showed that the fractionation introduced relatively little random noise ( Supplementary Fig. S6 ). The principal component analysis showed distinctive genome-wide expression profiles in different fractions with the fractionation as the first principal component (PC1, Supplementary Fig. S7 ). 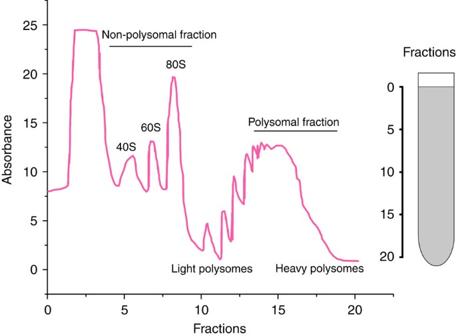Figure 3: Real-time optical density detection of the polysome fractions. Fractions were monitored using an ISCO UA-6 ultraviolet detector. The positions of 80S ribosomes, light polysomes and heavy polysomes, in the gradients are labelled. Two fractions, that is, non-polysomal fraction (corresponds to fraction 7–10) and polysomal fraction (corresponds to fraction 15–18) used in this study are indicated with arrows.xaxis: the fraction number (from fraction 1 to fraction 24);yaxis: the ultraviolet absorbance. Increases in polysome size by a single ribosome are indicated by secondary peaks in the up-slope of the broad polysome peak. Figure 3: Real-time optical density detection of the polysome fractions. Fractions were monitored using an ISCO UA-6 ultraviolet detector. The positions of 80S ribosomes, light polysomes and heavy polysomes, in the gradients are labelled. Two fractions, that is, non-polysomal fraction (corresponds to fraction 7–10) and polysomal fraction (corresponds to fraction 15–18) used in this study are indicated with arrows. x axis: the fraction number (from fraction 1 to fraction 24); y axis: the ultraviolet absorbance. Increases in polysome size by a single ribosome are indicated by secondary peaks in the up-slope of the broad polysome peak. Full size image Data analysis The gene expression data were normalized by robust spline normalization using the Lumi Bioconductor package [52] , implemented in the FlexArray software (genomequebec.mcgill.ca/FlexArray). Probe signals for 17,255 autosomal genes were assayed on the HumanRef-8 v3.0 Expression Beachip, and the expressions of 15,265 genes were detectable in the LCLs. The log 10 transformed ratio of normalized polysomal/non-polysomal signals was taken as the quantitative trait for the examination of the effect of exonic SNPs. The HapMap Phase 2 and Phase 3 genotyping data of these individuals were bulk-downloaded from the HapMap website (( http://www.hapmap.org/ ). The 1,000 genomes genotyping data were acquired from Dr Yun Li ( http://www.sph.umich.edu/csg/abecasis/MACH/download/1000G-2010-06.html ). Among the 38 individuals in our study, 9 individuals had no data from the 1000 Genomes Project. The genotypes of the missing 1,000 genomes SNPs of these 9 individuals were imputed based on the HapMap data using the MACH 1.0 software ( http://www.sph.umich.edu/csg/abecasis/MACH/index.html ). The 11.5% of SNPs with an imputation quality score <0.90 were discarded. Exonic SNPs were identified according to the SeattleSeq SNP Annotation ( http://snp.gs.washington.edu/SeattleSeqAnnotation/ ) based on dbSNP build 134. The cis -regulation of ribosomal distribution of gene mRNAs on the 22 autosomes by exonic SNPs was investigated. Quantitative trait association between the expression data and SNP genotype were tested using the Spearman rank correlation, as previously described for transcription data [53] . The workflow of this project is summarized in Fig.4 . 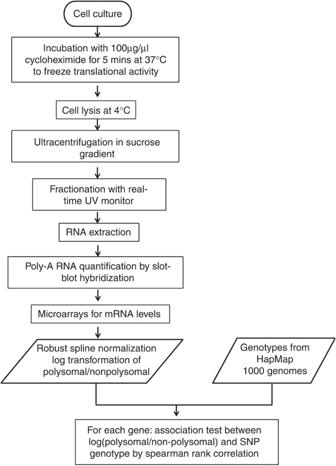Figure 4: Flowchart of the experimental approach for translationalcis-regulation in the human genome. The sedimentation velocity of mRNA–ribosomal complexes is taken as a proxy for mRNA translational efficiency. Figure 4: Flowchart of the experimental approach for translational cis- regulation in the human genome. The sedimentation velocity of mRNA–ribosomal complexes is taken as a proxy for mRNA translational efficiency. Full size image Ex vivo quantification of RPS26 protein The protein content in the total protein extract was measured in the LCLs of 36 of the CEU subjects and, after adjustment for specific mRNA level, compared among the three genotypes. Cells were washed with PBS and mixed with the appropriate volume of cell extraction buffer consisting of 98% TALON buffer, 1% protease inhibitor and 1% phenylmethylsulfonyl fluoride. Samples were subject to vortexing every 10 min for 10 s to ensure complete lysis, and after 30 min they were centrifuged at 20,000 g for 20 min. The supernatant was transferred to a clean tube and stored at −80 °C. Total protein concentration was determined using the Pierce BCA (bicinchoninic acid) Protein Assay Kit (Thermo Scientific, USA) and was used to dilute samples to the same concentration. Relative content of the target protein was measured by quantitative western blots. Rabbit RPS26 polyclonal antibody (ProteinTech Group, Illinois, USA) was diluted to 1:2,000 and mixed with 5% milk blocking solution (5 g of non-fat milk per 100 ml of tris buffered saline with tween). Mouse calnexin antibody (BD Biosciences, California, USA) at 1:2,000 dilution was used to measure the housekeeping gene control. Bands were visualized with the Western Lightning Chemiluminescence ECL plus detection kit (PerkinElmer, MA, USA). ImageJ software ( http://rsb.info.nih.gov/ij/index.html ) was used to compare the density of the RPS26 bands of the different samples for relative quantification. In each sample the density of the calnexin band (loading-control band) was used to scale the values for RPS26 protein. To assess translation, protein results were corrected for the amount of mRNA in each sample. In parallel to the protein extraction from the LCLs, RNA was also obtained using the RNeasy Plus Mini Kit (Qiagen, CA, USA). After reverse transcription, multiplex ligation-dependent probe amplification was used to measure the complementary DNA levels of RPS26 in all the samples. multiplex ligation-dependent probe amplification peaks were obtained in the ABI 310 Genetic Analyzer (Applied Biosystems, California, USA). The RPS26 signals were normalized using a probe set of the housekeeping microglobulin M 2 gene, whose expression was found to be the most invariant in the microarrays. Quantification of in vitro RPS26 protein translation Plasmid constructs containing different alleles of rs1131017 were made to study in vitro the effects of rs1131017 on translational efficiency. TA cloning was done using the pGEM vector (Promega, WI, USA). Each allele was constructed twice, each time with a different tag epitope: flag or myc . The linearized DNA plasmids were verified by Sanger sequencing. RNA from each allele construct was generated using an in vitro transcription kit (Ribomax Large Scale RNA Production–T7, Promega, WI, USA). The in vitro- produced DNAase-treated RNAs were purified using the RNeasy Plus Mini Kit (Qiagen). The Ribogreen RNA assay (Molecular Probes, OR, USA) was used to quantify the RNA samples. RT–PCR and Sanger sequencing were used to confirm the in vitro -produced RNAs. The in vitro synthesis of proteins in cell-free extracts was done in the Flexi rabbit reticulocyte lysate system (Promega, WI, USA). Western Blotting was used to quantify the RPS26 protein produced by the different alleles, as described above. Accession codes: Microarray data have been deposited in the NCBI Gene Expression Omnibus (GEO) database under accession code GSE46195 . How to cite this article: Li, Q. et al. Genome-wide search for exonic variants affecting translational efficiency. Nat. Commun. 4:2260 doi: 10.1038/ncomms3260 (2013).